Bod1 regulates protein phosphatase 2A at mitotic kinetochores Mitotic entry and progression require the activation of several mitotic kinases and the proper regulation and localization of several phosphatases. The activity and localization of each of these enzymes is tightly controlled through a series of specific activators, inhibitors and regulatory subunits. Two proteins, Ensa and Arpp-19, were recently identified as specific inhibitors of PP2A-B55 and are critical for allowing full activity of Cdk1/cyclin B and entry into mitosis. Here we show that Bod1, a protein required for proper chromosome alignment at mitosis, shares sequence similarity with Ensa and Arpp-19 and specifically inhibits the kinetochore-associated PP2A-B56 holoenzyme. PP2A-B56 regulates the stability of kinetochore-microtubule attachments by dephosphorylating several kinetochore proteins. Loss of Bod1 changes the balance of phosphorylation at kinetochores, causing defects in kinetochore function. Bod1, Ensa and Arpp-19 define a family of specific PP2A inhibitors that regulate specific PP2A holoenzymes at distinct locations and points in the cell cycle. To maintain genetic fidelity during cell division, sister chromatids must be segregated equally to each daughter cell. Biorientation and congression of chromosomes onto the metaphase plate is governed by the interaction of the mitotic spindle with kinetochores located at the centromere of each chromatid. This interaction must be regulated such that robust attachments persist only at sister chromatids, which are properly bioriented. Regulation of kinetochore function occurs largely by the antagonistic action of a number of kinases and phosphatases that localize to kinetochores during mitosis, changing the phosphorylation status, and therefore function, of many of the core structural components [1] . Although there has been some advance in describing the regulation of protein phosphatase 1 at the kinetochore [2] , [3] , [4] , very little is known about the direct substrates or the regulation of PP2A at the kinetochore. PP2A holoenzymes are composed of catalytic (C), scaffold (A) and regulatory (B) subunits. Specificity and activity of the holoenzyme is defined by the binding of the B regulatory subunit. There are 18 different B subunits that can be separated into three distinct families: the B (B55α, β, γ and δ), B′ (B56α, β, γ, δ and ε) and B′′′. The numerous isoforms of each allow 75 possible combinations of holoenzyme, enabling enormous heterogeneity and substrate specificity [5] . PP2A holoenzymes containing B56 regulatory subunits localize to the inner centromere and kinetochore during mitosis. PP2A-B56 has been associated with maintenance of sister chromatid cohesion [6] , regulation of kinetochore-microtubule attachment and is necessary for proper chromosome biorientation [7] . Association of PP2A-B56 with kinetochore components is known to be regulated in a phosphorylation-dependent manner [8] but to date no direct regulators of PP2A phosphatase activity at the kinetochore have been identified. Ensa and Arpp-19 are small, heat stable, proteins that specifically bind to and inhibit PP2A holoenzymes containing the B55 regulatory subunits (‘PP2A-B55’) during late G2 and enable mitotic entry. This temporal specificity is achieved through phosphorylation of Ensa and Arpp-19 by Greatwall kinase (Gwl) at a conserved serine that enables them to interact with and inhibit PP2A-B55 (refs 9 , 10 ). We recently identified Bod1 as a small kinetochore-associated protein required for mitotic chromosome congression [11] . Bod1 short interfering RNA (siRNA) depletion causes a loss of phosphorylation of MCAK, a microtubule depolymerase that modulates kinetochore-microtubule attachment and is required for correction of improper kinetochore-microtubule attachments. Here we demonstrate that Bod1 contains a regulatory motif, analogous to that found in ENSA and ARPP-19, that allows it to bind to and regulate PP2A-B56 activity in a phosphorylation-dependent manner. Loss of Bod1 from kinetochores hyperactivates the phosphatase resulting in loss of phosphoepitopes at the kinetochore and delocalization of Plk1 and Sgo1. Therefore, Bod1 is required to fine tune PP2A phosphatase activity at the kinetochore to ensure efficient chromosome congression and maintenance of chromatid cohesion. Bod1 interacts with and inhibits PP2A-B56 Bod1 shares a number of conserved residues with Ensa and Arpp-19 including an aspartate (D98; for clarity, we use the numbering from the Bod1 sequence to refer to Bod1, Ensa and Arpp-19), known to be critical for interaction of Ensa and Arpp-19 with PP2A-B55 ( Fig. 1a ). Similar to Ensa and Arpp-19, Bod1 is also a heat stable protein (S. Mochida, personal communication) and shares a comparable predicted disorder profile ( Supplementary Fig. S1 ). To establish an interaction between Bod1 and PP2A, we immunoprecipitated Bod1 from HeLa cells stably expressing Bod1-green fluorescent protein (GFP) and observed specific binding of the B56 regulatory subunit of PP2A, but not the B55 subunit ( Fig. 1b ). Sgo1, a protein necessary for proper centromere cohesion, also interacts with all PP2A-B56 isoforms at the kinetochore [6] and we observed Sgo1 co-immunoprecipitating with Bod1. We performed reciprocal experiments, immunoprecipitating endogenous B56δ ( Supplementary Fig. S2a ) or B56α ( Supplementary Fig. S2b ) and observed Bod1-GFP co-immunoprecipitating. Further, we were able to detect endogenous Bod1 in immunoprecipitations from a stably expressing B56α-GFP cell line ( Fig. 1c ). 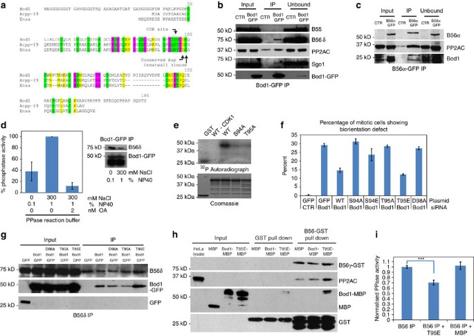Figure 1: Bod1 interacts with and inhibits PP2A-B56 and is regulated in a phosphorylation-dependent manner. (a) Alignment of Bod1 (NP_612378.1) with Arpp-19 (NP_006619.1) and Ensa (CAG38815.1). Conserved residues are in yellow, conserved hydrophilic and hydrophobic residues are in green and pink, respectively. (b,c) Bod1-GFP and B56α-GFP immunoprecipitates (IP), respectively, from STLC-arrested HeLa cells stably expressing Bod1-GFP or B56α-GFP. IPs were analysed by western blotting using antibodies against GFP, Bod1, B56δ, B56α, PP2A-C, Sgo1 and B55. (d) Bod1 IPs were incubated with phospho-PBIP1tide in the presence or absence of high concentrations of salt and detergent. Phosphate release was assayed using a malachite green phosphate detection kit,n=4. The ability of Bod1 to interact with PP2A-B56 under the indicated salt and detergent conditions was determined by immunoprecipitation. (e) Purified WT, S94A or T95A GST-Bod1 were incubated in buffer containing γ-32P ATP in the presence or absence of Cdk1/cyclin B. SDS–polyacrylamide gel electrophoresis-separated proteins were subjected to colloidal Coomassie staining and autoradiography. (f) HeLa cells were co-transfected with the indicated siRNA and plasmids expressing GFP alone or siRNA-resistant GFP-Bod1 variants as indicated. Forty-eight hours after transfection, cells were fixed and stained with 4',6-diamidino-2-phenylindole and tubulin markers and mitotic cells were scored for biorientation defects (100 cells per condition),n=3. (g) B56δ IPs from monastrol arrested cells transiently transfected with the indicated Bod1-GFP plasmids. IPs were analysed by western blotting for B56δ, Bod1 and GFP. (h) MBP, MBP-wtBod1 or MBP-T95E-Bod1 were incubated within vitro-reconstituted PP2A-B56 and analysed by western blotting for binding to the holocomplex. (i) Phosphate release from phospho-PBIP1 tide was measured after B56α-GFP IPs were incubated with buffer alone (n=12), MBP (n=6) or MBP-T95E-Bod1 (n=7), (***P<0.005, the Mann–WhitneyU-test). Error bars represent s.e.m. Figure 1: Bod1 interacts with and inhibits PP2A-B56 and is regulated in a phosphorylation-dependent manner. ( a ) Alignment of Bod1 (NP_612378.1) with Arpp-19 (NP_006619.1) and Ensa (CAG38815.1). Conserved residues are in yellow, conserved hydrophilic and hydrophobic residues are in green and pink, respectively. ( b , c ) Bod1-GFP and B56α-GFP immunoprecipitates (IP), respectively, from STLC-arrested HeLa cells stably expressing Bod1-GFP or B56α-GFP. IPs were analysed by western blotting using antibodies against GFP, Bod1, B56δ, B56α, PP2A-C, Sgo1 and B55. ( d ) Bod1 IPs were incubated with phospho-PBIP1tide in the presence or absence of high concentrations of salt and detergent. Phosphate release was assayed using a malachite green phosphate detection kit, n=4 . The ability of Bod1 to interact with PP2A-B56 under the indicated salt and detergent conditions was determined by immunoprecipitation. ( e ) Purified WT, S94A or T95A GST-Bod1 were incubated in buffer containing γ- 32 P ATP in the presence or absence of Cdk1/cyclin B. SDS–polyacrylamide gel electrophoresis-separated proteins were subjected to colloidal Coomassie staining and autoradiography. ( f ) HeLa cells were co-transfected with the indicated siRNA and plasmids expressing GFP alone or siRNA-resistant GFP-Bod1 variants as indicated. Forty-eight hours after transfection, cells were fixed and stained with 4',6-diamidino-2-phenylindole and tubulin markers and mitotic cells were scored for biorientation defects (100 cells per condition), n =3. ( g ) B56δ IPs from monastrol arrested cells transiently transfected with the indicated Bod1-GFP plasmids. IPs were analysed by western blotting for B56δ, Bod1 and GFP. ( h ) MBP, MBP-wtBod1 or MBP-T95E-Bod1 were incubated with in vitro -reconstituted PP2A-B56 and analysed by western blotting for binding to the holocomplex. ( i ) Phosphate release from phospho-PBIP1 tide was measured after B56α-GFP IPs were incubated with buffer alone ( n =12), MBP ( n =6) or MBP-T95E-Bod1 ( n =7), (*** P <0.005, the Mann–Whitney U -test). Error bars represent s.e.m. Full size image The above data suggest that Bod1 specifically interacts with PP2A-B56, suggesting that, like Ensa and Arpp-19, Bod1 might inhibit the catalytic activity of the PP2A holocomplex. To test this hypothesis, we incubated Bod1-GFP immunoprecipitates (IPs) with a phosphopeptide derived from the polo binding-domain (PBD) of PBIP1 (ref. 12 ) and measured released phosphate ion. Phosphatase activity associated with mitotic Bod1 IPs was low when assayed in low salt/detergent buffer but increased in a high salt/detergent buffer that dissociated Bod1 from PP2A-B56 ( Fig. 1d ). This activity was inhibited by 2 nM okadaic acid, suggesting that the activity was PP2A dependent ( Fig. 1d ). Similar results were observed in IPs from asynchronously growing cells, although overall phosphatase activity associated with these precipitates was reduced compared with precipitates from mitotic cells ( Supplementary Fig. S2c ). Overall, these data demonstrate that Bod1 associates with PP2A-B56 and inhibits its catalytic activity. Ensa and Arpp-19 are phosphorylated by Gwl at S99 adjacent to the conserved D98. This Gwl site is missing in Bod1, but a potential Cdk1 kinase site is present at T95 ( Fig. 1a ). Recombinant Bod1 was phosphorylated in vitro by purified Cdk1/cyclin B and phosphorylation was substantially reduced in Bod1 S94A or T95A mutants, suggesting that both residues may be phosphorylated in vitro ( Fig. 1e ). To determine whether these sites, or the conserved adjacent aspartate (D98), were required for Bod1 function, we depleted endogenous Bod1 by siRNA in HeLa cells, expressed various siRNA-resistant Bod1-GFP mutants and then determined whether each mutant rescued defects in biorientation ( Fig. 1f ). Expression of wtBod1-GFP partially rescued the biorientation defect; presence of the GFP tag likely prevented full rescue. Only the T95E phosphomimetic mutant rescued as effectively as wild type suggesting that phosphorylation at T95 is required for Bod1 function. S94A, T95A and D98A mutants all failed to efficiently rescue Bod1 function in this assay. Immunoprecipitation experiments with these mutants demonstrated increased binding of the T95E mutant to B56δ and decreased binding of the T95A and D98A mutants ( Fig. 1g ). We next assessed whether recombinant Bod1 could interact with B56 in vitro . Glutathione S -transferase (GST)-Bod1 alone could not pull down recombinant B56δ ( Supplementary Fig. S2d ); hence, we tested the ability of Bod1 to bind to the PP2A-B56 holoenzyme. We were unable to efficiently produce a fully recombinant holoenzyme ( Supplementary Fig. S2e ); instead, we produced an in vitro -reconstituted PP2A-B56 holocomplex using B56γ-GST to pull out PP2A-A/C dimers from mitotic HeLa lysates. Consistent with our functional and immunoprecipitation results, only the T95E mutant bound efficiently to the reconstituted PP2A-B56 ( Fig. 1h ). Binding of recombinant maltose binding protein (MBP)-T95E-Bod1 to immunoprecipitated GFP-B56α holoenzyme ( Supplementary Fig. S2f ) also resulted in reduced phosphatase activity ( Fig. 1i ). This reduction in activity was specific to Bod1 as addition of equimolar amounts of MBP did not affect activity. Together, these results suggest that T95 phosphorylation and D98 are essential for the function of Bod1 and inhibition of PP2A-B56. Bod1 maintains localization of Sgo1 and Plk1 at kinetochores PP2A-B56 and Sgo1 localize to centromeres during mitosis and protect sister chromatid cohesion before anaphase onset [6] , [13] . We therefore assessed the effect of Bod1 depletion on PP2A-B56 and Sgo1 localization and function. Bod1 depletion resulted in increased B56α and reduced Sgo1 at centromeres ( Fig. 2a–d ). We observed no change in Sgo1 protein levels ( Fig. 2e ), indicating that Sgo1 is delocalized in Bod1-depleted cells but is not degraded. Bod1 depletion also resulted in loss of sister chromatid cohesion and premature separation of sister chromatids ( Fig. 2f,g ). Live cell imaging of CENP-B-GFP-expressing cells showed that Bod1 depletion causes a cohesion defect that is indistinguishable from depletion of Sgo1 (ref. 14 ) ( Fig. 2f ). These data suggest that Sgo1 must be correctly targeted to centromeres to properly maintain centromeric cohesion and that Sgo1 localization and function critically depend on Bod1. 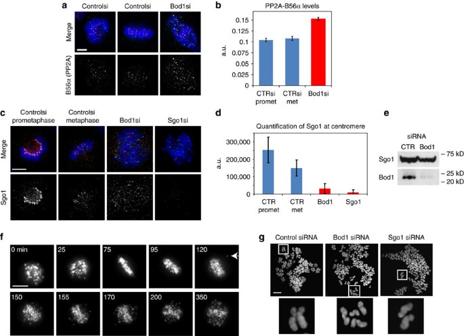Figure 2: Bod1 is required for sister chromatid cohesion. (a) Representative images of HeLa cells that were transfected with control or Bod1 siRNA and prepared for IF 48 h after transfection. Cells were stained using an anti-centromere antibody (red) and anti-B56α antibody (green). Chromosomes were stained with 4',6-diamidino-2-phenylindole (blue). (b) Quantitation of B56α levels at centromere/kinetochore of control and Bod1 siRNA-transfected cells (3 replicates; in each replicate 10 cells (>1,000 kinetochores) measured per condition). (c,d) Representative images and quantitation of Sgo1 levels in HeLa cells transfected with control, Bod1 or Sgo1 siRNA. (e) WB showing Sgo1 and Bod1 levels in HeLa cells transfected with control or Bod1 siRNA (2 replicates; in each replicate 2 cells (>50 kinetochores) measured per condition). (f) Selected time points from a time-lapse series of HeLa cells co-transfected with GFP-CENP-B and Bod1 siRNA. Arrowhead indicates first frame with a detectable single sister chromatid off the metaphase plate. (g) Chromosome spreads of nocodazole-arrested HeLa cells transfected with control, Bod1 or Sgo1 siRNA. Scale bars, 5 μm. Error bars represent s.e.m. Figure 2: Bod1 is required for sister chromatid cohesion. ( a ) Representative images of HeLa cells that were transfected with control or Bod1 siRNA and prepared for IF 48 h after transfection. Cells were stained using an anti-centromere antibody (red) and anti-B56α antibody (green). Chromosomes were stained with 4',6-diamidino-2-phenylindole (blue). ( b ) Quantitation of B56α levels at centromere/kinetochore of control and Bod1 siRNA-transfected cells (3 replicates; in each replicate 10 cells (>1,000 kinetochores) measured per condition). ( c , d ) Representative images and quantitation of Sgo1 levels in HeLa cells transfected with control, Bod1 or Sgo1 siRNA. ( e ) WB showing Sgo1 and Bod1 levels in HeLa cells transfected with control or Bod1 siRNA (2 replicates; in each replicate 2 cells (>50 kinetochores) measured per condition). ( f ) Selected time points from a time-lapse series of HeLa cells co-transfected with GFP-CENP-B and Bod1 siRNA. Arrowhead indicates first frame with a detectable single sister chromatid off the metaphase plate. ( g ) Chromosome spreads of nocodazole-arrested HeLa cells transfected with control, Bod1 or Sgo1 siRNA. Scale bars, 5 μm. Error bars represent s.e.m. Full size image Localization of Plk1 kinase during mitosis is dependent on both PP2A and Sgo1 (refs 7 , 15 ). Plk1 localization also changes throughout mitosis in a manner dependent on Plk1 phosphorylation of PBD in substrates that then serve as binding sites for Plk1 (refs 16 , 17 ). We predicted that loss of Bod1 should result in the loss of PP2A-B56 inhibition at kinetochores, and thus inappropriate dephosphorylation of centrosome- and kinetochore-associated PBDs. Indeed, phosphorylation of PBIP1, a known kinetochore substrate and binding site for Plk1 (ref. 18 ) that contains the sequence used in our in vitro phosphatase assays ( Fig. 1d ), was reduced fourfold in Bod1-depleted cells, removing at least one targeting site for Plk1 ( Fig. 3a–d ). Consistent with this, Bod1 depletion caused loss of Plk1 from kinetochores ( Fig. 3e,f ). Loss of PBIP phosphorylation and Plk1 localization was not due to increased tension across kinetochore pairs as the interkinetochore distance in Bod1-depleted cells was reduced even compared with control prometaphase cells ( Fig. 3h,i ), a phenotype that is identical to that observed after Sgo1 depletion [14] ( Fig. 3i ). These changes occurred without detectable effect on Plk1 activation or kinase activity ( Fig. 3j,k ). Nonetheless, Plk1 function was compromised: Bod1-depleted cells were hypersensitive to the Plk1 inhibitor BI 2536, generating monopolar spindles at lower concentrations of the drug than control cells ( Fig. 3l ). 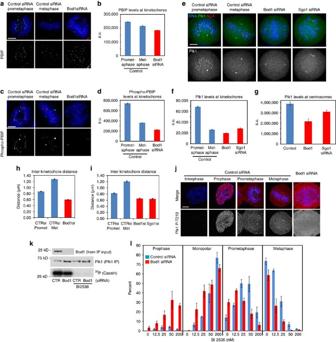Figure 3: Plk1 is delocalized from kinetochores in Bod1-depleted cells. (a,b) Representative images and quantitation of PBIP1 localization at kinetochores of control and Bod1 siRNA-transfected HeLa cells (3 replicates; in each replicate 10 cells (>1,000 kinetochores) measured per condition). (c,d) Representative images and quantitation of phospho-PBIP1 localization at kinetochores of control and Bod1 siRNA-transfected HeLa cells (3 replicates; in each replicate 10 cells (>1,000 kinetochores) measured per condition). (e–g) Representative images and quantitation of Plk1 levels at kinetochores and centrosomes in control, Bod1 or Sgo1 siRNA-transfected HeLa cells (2 replicates; in each replicate:f, 4 cells (50 kinetochores) per condition;g, 10 cells (20 centrosomes) per condition). (h,i), Interkinetochore distance between identifiable sister pairs of data fromdandf, respectively (h,n=300 sister pairs from 10 cells per condition;i,n=120–160 sister pairs from five cells per condition). (j) Representative images of anti-Plk1 phospho-T210 staining of HeLa cells transfected with control or Bod1 siRNA. (k) Upper panel: WB of Bod1 levels in control and Bod1 siRNA-transfected cells. Middle panel: WB of Plk1 immunoprecipitated from cell lysates. Bottom panel: autoradiograph of [γ-32P] incorporation into casein after incubation with Plk1 IP±Plk1 inhibitor BI 2536. (l) Mitotic profile of control and Bod1 siRNA-transfected HeLa cells 1 h after release from an 18-h incubation with Cdk1 inhibitor RO-3306 into the indicated concentrations of BI 2536 (100 cells per condition/drug concentration),n=3. Scale bars, 5 μm. Error bars represent s.e.m. Figure 3: Plk1 is delocalized from kinetochores in Bod1-depleted cells. ( a , b ) Representative images and quantitation of PBIP1 localization at kinetochores of control and Bod1 siRNA-transfected HeLa cells (3 replicates; in each replicate 10 cells (>1,000 kinetochores) measured per condition). ( c , d ) Representative images and quantitation of phospho-PBIP1 localization at kinetochores of control and Bod1 siRNA-transfected HeLa cells (3 replicates; in each replicate 10 cells (>1,000 kinetochores) measured per condition). ( e – g ) Representative images and quantitation of Plk1 levels at kinetochores and centrosomes in control, Bod1 or Sgo1 siRNA-transfected HeLa cells (2 replicates; in each replicate: f , 4 cells (50 kinetochores) per condition; g , 10 cells (20 centrosomes) per condition). ( h , i ), Interkinetochore distance between identifiable sister pairs of data from d and f , respectively ( h , n =300 sister pairs from 10 cells per condition; i , n =120–160 sister pairs from five cells per condition). ( j ) Representative images of anti-Plk1 phospho-T210 staining of HeLa cells transfected with control or Bod1 siRNA. ( k ) Upper panel: WB of Bod1 levels in control and Bod1 siRNA-transfected cells. Middle panel: WB of Plk1 immunoprecipitated from cell lysates. Bottom panel: autoradiograph of [γ- 32 P] incorporation into casein after incubation with Plk1 IP±Plk1 inhibitor BI 2536. ( l ) Mitotic profile of control and Bod1 siRNA-transfected HeLa cells 1 h after release from an 18-h incubation with Cdk1 inhibitor RO-3306 into the indicated concentrations of BI 2536 (100 cells per condition/drug concentration), n =3. Scale bars, 5 μm. Error bars represent s.e.m. Full size image Bod1 is required for Plk1-dependent centrosome maturation Plk1 is required at multiple locations and times during cell cycle progression, and in particular for proper centrosome maturation during mitotic entry and establishment of a bipolar spindle [19] , [20] , [21] , [22] . To further characterize the cause of defects in Plk1 function in Bod1-depleted cells, we examined mitotic spindles and observed reduced Plk1 localization at the centrosomes of these cells ( Fig. 3e,g ). Downstream centrosomal targets of Plk1, including γ-tubulin, sSgo1 and cenexin [23] , [24] , [25] were also delocalized ( Fig. 4a–f ) consistent with the reduction of Plk1 function in Bod1-depleted cells. These pleiotropic effects on Plk1 function explain our original observation of spindle length and organizational defects in Bod1-depleted cells [11] . Taken together, these results suggest that Bod1 regulates Plk1 function through inhibition of PP2A-B56 at both spindle poles and kinetochores of mitotic cells. 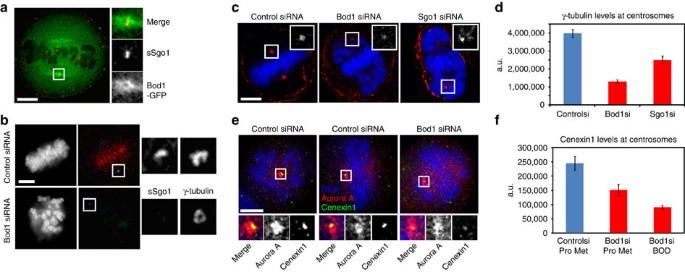Figure 4: Plk1 substrates are delocalized from centrosomes of Bod1-depleted HeLa cells. (a) Localization of sSgo1 (red) and Bod1-GFP (green) at centrosomes of HeLa cells. (b) Representative images of sSgo1 localization to centrosomes in control and Bod1 siRNA-transfected HeLa cells. In merged image, Sgo1 is in red and γ-tubulin in green. (c,d) Representative images and quantitation of γ-tubulin levels at centrosomes in control, Bod1 or Sgo1 siRNA-transfected HeLa cells. DNA (blue), γ-tubulin (red) (3 replicates; in each replicate 20 cells (40 centrosomes) measured per condition). (e) Representative images of cenexin1 levels at the centrosome of control siRNA cells during prometaphase and metaphase and a mitotic cell depleted of Bod1. DNA is in blue, aurora A in red and cenexin1 in green (f) Quantitative analysis of cenexin1 levels in HeLa cells transfected with control or Bod1 siRNA (2 replicates; in each replicate 10–20 cells (20–40 centrosomes) measured per condition). Scale bars, 5 μm. Error bars represent s.e.m. Figure 4: Plk1 substrates are delocalized from centrosomes of Bod1-depleted HeLa cells. ( a ) Localization of sSgo1 (red) and Bod1-GFP (green) at centrosomes of HeLa cells. ( b ) Representative images of sSgo1 localization to centrosomes in control and Bod1 siRNA-transfected HeLa cells. In merged image, Sgo1 is in red and γ-tubulin in green. ( c , d ) Representative images and quantitation of γ-tubulin levels at centrosomes in control, Bod1 or Sgo1 siRNA-transfected HeLa cells. DNA (blue), γ-tubulin (red) (3 replicates; in each replicate 20 cells (40 centrosomes) measured per condition). ( e ) Representative images of cenexin1 levels at the centrosome of control siRNA cells during prometaphase and metaphase and a mitotic cell depleted of Bod1. DNA is in blue, aurora A in red and cenexin1 in green ( f ) Quantitative analysis of cenexin1 levels in HeLa cells transfected with control or Bod1 siRNA (2 replicates; in each replicate 10–20 cells (20–40 centrosomes) measured per condition). Scale bars, 5 μm. Error bars represent s.e.m. Full size image Co-depletion of Bod1 and PP2A-B56 rescues Plk1 localization If Bod1 depletion relieves inhibition of PP2A-B56 and this hyperactive enzyme dephosphorylates PBDs and delocalizes Plk1, then specific depletion or inhibition of PP2A-B56 should restore Plk1 localization. siRNA targeting all B56 subunits [7] in Bod1-depleted cells rescued Plk1 localization to kinetochores ( Fig. 5a,b ; Supplementary Fig. S3a ), consistent with our model that Bod1 is required to inhibit PP2A-B56. Recovery of Sgo1 was not observed after co-depletion of Bod1 and B56 subunits ( Supplementary Fig. S3b ), which is consistent with previous reports showing that PP2A-B56 is required for Sgo1 localization to kinetochores [6] . These results suggest that Bod1 modulates Plk1 localization by directly regulating PP2A-B56 function. Moreover, this result may explain why depletion of B56 subunits causes an increase in Plk1 localization to kinetochores [7] . 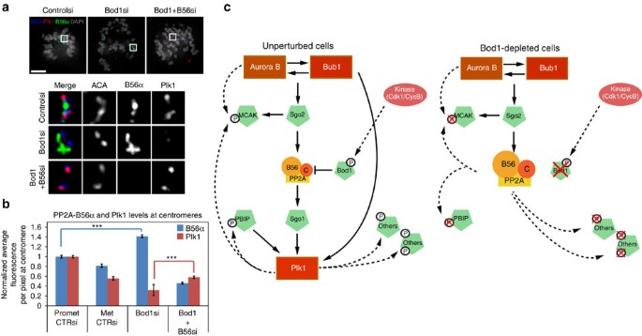Figure 5: Co-depletion of PP2A with Bod1 rescues Plk1 localization. (a) HeLa cells were transfected with control or Bod1 siRNA, or co-transfected with PP2A and Bod1 siRNA. Forty-eight hours after transfection, cells were prepared for IF and stained for Plk1 (red), B56α (green) and anti-centromere antibody (blue). Chromosomes were detected with 4',6-diamidino-2-phenylindole. Upper panels show representative images. Lower panels show enlargement of the areas bounded by a white box in the upper panels. (b) Quantification of B56α and Plk1 fluorescence signal at centromeres of cells transfected as ina(3 replicates; in each replicate 10 cells (>1,000 kinetochores) measured per condition). ***P<0.001, Student’st-test). (c) Model for recruitment and phosphorylation of selected proteins to kinetochores under normal conditions (left) and in Bod1-depleted cells (right). Solid black arrows show a requirement for recruitment. Dashed black lines demonstrate phosphorylation/dephosphorylation events. Scale bars, 5 μm. Error bars represent s.e.m. Figure 5: Co-depletion of PP2A with Bod1 rescues Plk1 localization. ( a ) HeLa cells were transfected with control or Bod1 siRNA, or co-transfected with PP2A and Bod1 siRNA. Forty-eight hours after transfection, cells were prepared for IF and stained for Plk1 (red), B56α (green) and anti-centromere antibody (blue). Chromosomes were detected with 4',6-diamidino-2-phenylindole. Upper panels show representative images. Lower panels show enlargement of the areas bounded by a white box in the upper panels. ( b ) Quantification of B56α and Plk1 fluorescence signal at centromeres of cells transfected as in a (3 replicates; in each replicate 10 cells (>1,000 kinetochores) measured per condition). *** P <0.001, Student’s t -test). ( c ) Model for recruitment and phosphorylation of selected proteins to kinetochores under normal conditions (left) and in Bod1-depleted cells (right). Solid black arrows show a requirement for recruitment. Dashed black lines demonstrate phosphorylation/dephosphorylation events. Scale bars, 5 μm. Error bars represent s.e.m. Full size image We have identified Bod1 as a regulator of PP2A-B56 function at kinetochores. Together with Ensa and Arpp-19, Bod1 defines a new family of protein PP2A inhibitors that inhibit phosphatase activity at specific times and locations during mitosis. These inhibitors share a conserved PP2A-B subunit-binding mechanism that depends on the phosphorylation of serine or threonine adjacent to a highly conserved aspartate that is critical for binding of the PP2A-B subunit. All of these inhibitors are heat stable and share a pattern of disordered and folded regions across their sequence. Our data indicate that Bod1, the newest member of this family, specifically inhibits PP2A-B56 at mitotic kinetochores and centrosomes. Just as protein phosphatase 1 activity has to be precisely balanced against the activity of various kinases such as Aurora B during mitosis by inhibitor-2 (refs 26 , 27 , 28 ), it is now clear that PP2A activity is also carefully regulated by the family of novel inhibitors Ensa, Arpp-19 and Bod1. In common with endosulphines Arpp-19 and Igo1 (refs 9 , 29 ), recombinant Bod1 is a relatively poor inhibitor of PP2A, whereas Bod1 from cell lysates is a more potent inhibitor of its associated PP2A ( Fig. 1d,i ; Supplementary Fig. S2c ). This suggests that additional post-translational modifications of Bod1 may be required for full inhibition of PP2A-B56. Alternatively, Bod1 may only efficiently interact with pools of PP2A-B56 containing specific post translational modifications or additional accessory factors. Depletion of Bod1 causes a range of defects all of which are consistent with increased levels of PP2A activity. Figure 5c shows how inhibition of PP2A-B56 by Bod1 at kinetochores might modulate function and localization of a number of kinetochore proteins. Loss of Bod1 relieves inhibition of PP2A-B56 and delocalizes Plk1 from kinetochores, probably through loss of phosphorylation of several PBD-containing kinetochore components. Overall, this results in stabilization of kinetochore-microtubule contacts—Bod1-depleted cells have elevated levels of syntelic attachments and fail to fully recover from a monastrol arrest [11] . Indeed, removing the PP2A-B56 subunit by RNA interference depletion produces the opposite effect—Plk1 targeting to kinetochores increases and kinetochore-microtubule interactions are destabilized [7] . Bod1 depletion very likely reduces phosphorylation of Sgo1, which is critical for proper Sgo1 localization and function in multiple species [30] , [31] . We note that although PP2A-B56 interacts with Sgo1 and is required for its localization [6] , [32] , loss of PP2A-B56 inhibition through Bod1 depletion interferes with Sgo1 localization and causes a cohesion defect. Two recent papers [33] , [34] have described ‘cohesion fatigue’ resulting in uncoordinated scattering of sister chromatids as a consequence of an extended metaphase delay. Although poorly understood, it will be interesting to determine how this phenomenon compares mechanistically with direct loss of cohesion upon the loss of Sgo1. Upon loss of Bod1, we also observe centrosomal defects—delocalization of Plk1 and associated proteins that require Plk1 for their localization. These pleotropic effects highlight the importance of PP2A activity and its modulation by Bod1 and its relatives in different locations in the cell. Bod1 has recently been identified as a member of the SET1 methyltransferase complex [35] . It will be interesting to determine whether this complex has any role in mitosis, or, as Bod1 and PP2A-B56 are expressed in many different cell types, including terminally differentiated cells like neurons, whether Bod1 works as a modulator of PP2A-B56 in other regulatory pathways through this complex or others. Cell lines and cell culture HeLa S3 cells were maintained in EMEM (Lonza) and supplemented with 10% fetal calf serum, 2 mM L -glutamine, 100 U ml −1 penicillin and 100 μg ml −1 streptomycin. A cell line stably expressing Bod1-GFP was generated using the HeLa Flp-In cell line described in Klebig et al . [36] , (a kind gift from Patrick Meraldi), maintained in the media described above with an additional 200 μg ml −1 hygromycin. B56α-GFP stable cell lines (a kind gift from Tarun Kapoor) were maintained as described above with an additional 700 nM puromycin. Cells lines were maintained at 37 °C with 5% CO 2 in a humidified incubator. HeLa cells were transfected with plasmid DNA and siRNA oligo duplexes using Lipofectamine 2000 (Invitrogen). Medium GC control siRNA was supplied by Invitrogen. Bod1 siRNA 5′-GCCACAAAUAGAACGAGCAAUUCAU-3′ was as described [11] . Pooled Sgo1 siRNA targeted 5′-CCUGCUCAGAACCAGGAAATT-3′ and GAGGGGACCCUUUUACAGATT were as described [37] . The PP2A-B56 siRNA pool targeted B56α (PPP2R5A), 5′-GCUCAAAGAUGCCACUUCA-3′; B56β (PPP2R5B), 5′-CGCAUGAUCUCAGUGAAUA-3′; B56γ (PPP2R5D), 5′-GGAUUUGCCUUACCACUAA-3′; B56δ (PPP2R5D), 5′-UCCAUGGACUGAUCUAUAA-3′; and B56ε(PPP2R5E), 5′-UUAAUGAACUGGUGGACUA-3′ were as described [7] . Unless otherwise indicated nocodazole was used at 100 ng ml −1 , monastrol at 100 nM, RO 3,306 at 9 μM, BI 2,536 at 12.5–200 nM and MG132 at 10 μM. Microscopy and antibodies Time-lapse imaging and fluorescence microscopy was performed as described [11] . All images were stored and manipulated using OMERO or Photoshop (Adobe). Antibodies and their respective applications (western blot (WB) and immunofluorescence (IF)): rabbit anti-Bod1 (Porter et al . [11] ) (WB) and mouse anti-B56α (BD Biosciences) (IF) were used at 1:100. Mouse anti-Sgo1 (Abcam; WB, IF), mouse anti-Aurora A (Sigma; IF), rabbit anti-PBIP1 (MLF1IP; Rockland; IF) and rabbit anti-Cenexin1/ODF2 (Abcam; IF) were used at 1:200. Mouse anti-Plk1 (Upstate; WB, IF), rabbit anti-pT78-PBIP1 (Abcam; IF), mouse anti-B56α (Abcam; WB), mouse anti-B56δ (Abcam; WB) and rabbit anti-γ-tubulin (Abcam; IF) were used at 1:500. Human anti-centromere autoantisera (ACA), (a kind gift from Sara Marshall, Ninewells Hospital, Dundee; IF), mouse anti-PP2Ac (Millipore, 1D6; WB) and mouse anti-pT210-Plk1 (BD Biosciences; IF) were used at 1:1,000. Mouse anti-GAPDH (Abcam; WB) was used at 1:3,000. Goat anti-PP2A-A (Santa Cruz; WB) was used at 1:5,000. Mouse anti-MBP (NEB; WB) was used at 1:20,000. All fluorescently labelled secondary antibodies were obtained from Jackson ImmunoResearch Laboratories. Quantification of IF images Fluorescence intensity of signals at centromeres/kinetochores was calculated in one of two ways: first, 10 × 10 pixel boxes were manually placed over centromeres and the summed pixel values of a given channel calculated. Another 10 × 10 box was placed adjacent to this to calculate background signal, which was then subtracted from the centromere signal. Thirty to forty centromeres were chosen per cell. Alternatively, using an application written in Matlab (The Mathworks) interacting with an OMERO server [38] , centromeres were identified automatically from deconvolved three-dimensional (3D) image stacks by applying Otsu thresholding to the anti-centromere antibody channel and generating 3D masks for individual centromeres. The perimeter of each mask was then expanded by 2–4 pixels to ensure coverage of the kinetochore and innercentromeric region. The summed fluorescent intensity and average intensity/pixel within the mask region was calculated for the other channels (including subtraction of the background signal). Manual identification and segmentation of clearly identifiable individual centromeres using Otsu thresholding indicated a maximum size of 750 pixels per centromere. This cutoff was applied to the automatic segmentation so only 3D objects smaller than 750 pixels were included in the summed analysis. Objects above this size were assumed to be multiple centromeres that the Otsu thresholding could not segment into individual bodies. Using this method, we were routinely able to identify ~80–100 individual centromeres per HeLa cell. For any given experiment, at least 10 cells were analysed per condition and experiments were repeated at least three times. Immunoprecipitation S-Tityl- L -cysteine (STLC)-arrested Bod1-GFP cells were lysed in lysis buffer (20 mM Tris acetate pH 7.5, 1 mM EGTA, 1 mM EDTA, 10 mM Na-β-glycerophosphate, 5 mM Na-pyrophosphate, 1 mM Na-orthovanadate, 50 mM NaF, 1 μM microcystin, 0.27 M sucrose, 0.01% Triton-X-100, 1 × complete protease inhibitors) with three to four rounds of freeze fracturing and immunoprecipitated using GFP-Binder (Chromotek), or with anti-B56α/δ antibody conjugated to protein-G sepharose. Phosphatase assay Bod1-GFP was immunoprecipitated as above, beads washed twice in PPase reaction buffer (50 mM HEPES, 1 mM dithiothreitol (DTT), 1 mM EDTA and 0.1% NP40), split into two equal fractions and resuspended in PPase reaction buffer with or without 1% NP40 and 300 nM NaCl. P-PBIPtide (6 mM) (ref. 12 ) CDPPLHS[p]TAIYADEE was added and incubated for 45 min at 30 °C. Phosphate release was measured using a Malachite Green Phosphate Detection kit (R&D Systems) as per the manufacturer’s instructions. STLC-arrested B56α-GFP cells were lysed and immunoprecipitated as above, except phosphatase inhibitors were excluded. The IP was split into equal fractions and incubated with buffer alone, 50 pmol MBP-T95E-Bod1 or 50 pmol MBP for 1 h followed by a single wash with PPase reaction buffer. Beads were resuspended in PPase reaction buffer ±2 nM okadaic acid. Phosphate released from PBIPtide was measured as above. PP2A-specific phosphate release was measured as activity inhibited by 2 nM okadaic acid. Generation of recombinant PP2A–B56γ holoenzyme The following expression constructs were used: PP2A-A-GST, PP2A-C(D88N)-GST, B56γ3Δ29-GST [39] (a kind gift from Wenqing Xu); GST-B56δ, GST-Bod1, GST, MBP-Bod1 MBP-T95E-Bod1 and MBP (this paper). Constructs were expressed and purified from BL21 cells. If applicable, the GST-Tag was cleaved with PreScission Protease (GE Healthcare) or TEV Protease (Promega). Initially, 200 pmol of Bod1-GST was conjugated to glutathione-separose and incubated with individual PP2A components (PP2A-A, PP2A-C(D88N) and B56δ), but no specific binding was observed. Alternatively, 200 pmol B56γ3Δ29-GST or GST were coupled to glutathione-sepharose and incubated with mitotic HeLa cell lysates to co-precipitate free cellular PP2A-C/A heterodimers. The holocomplex was washed with pull-down buffer (20 mM Tris–HCl, 20 mM NaCl, 10% glycerol, 1 mM EGTA, 1 mM DTT, Complete protease inhibitors (Roche) and 0.1% Triton-X), and then incubated with 100 pmol MBP, MBP-Bod1 or MBP-T95E-Bod1. The protein complexes were washed with interaction buffer (same as pull-down buffer but 0.5% Triton-X) and analysed by WB. Full scans of WBs are provided in Supplementary Fig. S4 . Cdk1 and Plk1 kinase assays Plk1 kinase immunoprecipitated from lysates prepared from nocodazole-arrested HeLa lysates, which had been transfected with control or Bod1 siRNA using anti-Plk1 antibody conjugated to Affi-prep Protein A. Plk1-bound beads were incubated with 5 μg casein in TADB (6.7 mM Tris–HCl pH 7.5, 13 μM EGTA, 2 mM DTT), IB (10 mM Na 2 HPO 4 , pH 7.4, 100 mM KCl, 1 mM MgCl 2 ) and magnesium/ATP cocktail (27.5 mM MgCl 2 , 0.183 mM ATP, 4 mM 3-( N -morpholino) propanesulfonic acid pH7.2, 9.17 mM β-glycerolphosphate, 1.83 mM EGTA, 0.37 mM sodium orthovanadate, 0.37 mM DTT) and 10 μCi [γ- 32 P]ATP for 30 min at 30 °C, ±200 nM BI 2536. Samples were separated on a 4–12% SDS–polyacrylamide gel electrophoresis, transferred to a nitrocellulose membrane and exposed to autoradiography or probed using anti-Plk1 or Bod1 antibodies. Cdk1/cyclin B (100 ng; Millipore) was mixed with TADB, IB and Mg/ATP cocktail and incubated for 30 min at 30 °C. [γ- 32 P]ATP (10 μCi) and 300 ng GST-Bod1 was then added and incubated for a further 30 min at 30 °C. Samples were separated on a 4–12% SDS–polyacrylamide gel electrophoresis gel, and the gel was dried and exposed to autoradiography. Chromosome spreads Chromosome spreads were performed as described [40] . Briefly, siRNA-transfected HeLa cells were incubated with 100 ng ml −1 nocodazole for 18 h. Following a gentle mitotic shake off, cells were incubated for 5 min in 40% media 60% water at room temperature, centrifuged and fixed in 1 ml fixative (3:1 methanol:acetic acid). Chromosomes were dropped onto coverslips preheated on a gradient heat block at 25–65 °C and dried until grainy. Chromosomes were stained using 4',6-diamidino-2-phenylindole. How to cite this article: Porter, I. M. et al . Bod1 regulates protein phosphatase 2A at mitotic kinetochores. Nat. Commun. 4:2677 doi: 10.1038/ncomms3677 (2013).